Anisotropy governs strain stiffening in nanotwinned-materials 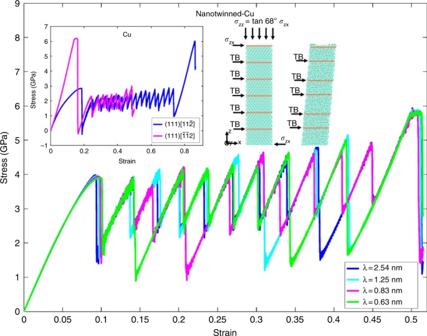Fig. 1 Stress-strain curves of single crystalline and nanotwinned-Cu, and simulation set-ups for molecular dynamics simulations on nanotwinned samples. Simulated stress-strain relations of nanotwinned-Cu samples with twin thickness varying fromλ= 0.63 nm to 2.54 nm. The strength of the material and the tangent of the strain stiffening part are the same for samples with different twin boundary (TB) spacings. The simulation set-ups are shown in the right inset of the figure. The nantwinned-Cu super-cell is subjected to both shear and compressive loading similar to the Vickers indentation experiments. The compression to shear ratio is fixed at a constant value of tan (68°). The left inset presents the stress-strain curves for a shear loading of a single crystalline Cu along hard (111)\([\bar 1\bar 12]\)and weak (111)\([11\bar 2]\)shear directions. Different slopes of the curves confirm the anisotropic behavior of Cu crystal similar to covalent-bonding materials All data generated and analyzed during this study are included in this published article.